Reply to: Questioning whether the IgM Fc receptor (FcμR) is expressed by innate immune cells 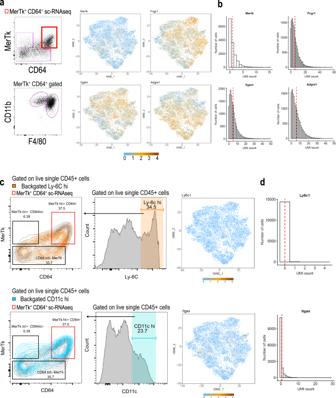Fig. 1: Discordance in flow cytometric protein data and scRNAseq read counts. aFlow cytometry dot plots (left) illustrate the population of MerTk+CD64+(bold red gate) tumor mononuclear phagocytes (TMP) that were FACS-sorted for scRNAseq (top left), and this populations CD11b and F4/80 expression (bottom left). The corresponding transcript data for the markers shown in the flow plots, which was obtained from scRNAseq analysis, is overlaid on t-SNE plots for each of the four genes that encode those markers; Mertk (MerTk), Fcgr1 (CD64), Itgam (CD11b), and Adgre (F4/80) (Right). These t-SNE represent cell clusters from FACS-sorted TMP isolated from B16 melanoma tumors growing inFcmr+/+andFcmr−/−mice. Gene expression is overlaid on these tSNEs to highlight differential read counts for each of the four genes, where a UMI of 0 is illustrated in blue.bHistograms illustrating the distributions of raw UMI counts per cell for those same four genes (Mertk,Fcgr1,Itgam, andAdgre) which were stained at the protein level during FACS-sorting of TMP. Mean count values are denoted by a vertical red dashed line.candd(Left) The bicolor contour plots illustrate surface receptors Ly-6c and CD11c backgated from histogram plots (middle), where the Ly-6chiis gated in orange (top) and the CD11chiis gated in blue (bottom). Apparent from the backgating (left), both surface receptors Ly-6c (Ly6c1) and CD11c (Itgax) are expressed at the protein level on the TMP that were sorted for scRNAseq. (Right) tSNE expression-overlaid plots forLy6c1(top right) andItgax(bottom right) show zero and near zero cells with transcript for these receptors. UMI of 0 is illustrated in blue.dHistograms illustrating the distribution of UMI forLy6c1andItgax, as inbabove. 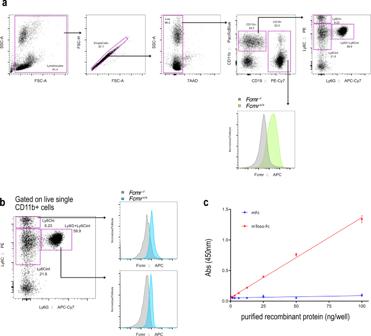Fig. 2: Fcmr is expressed in classical monocyte and neutrophil innate-immune cells. a(Top) Gating schematic for peripheral blood staining implementing an in-house anti-mouse-Fcmr antibody. (Bottom right) Histogram overlay of Fcmr staining of peripheral blood B cells inFcmr+/+(green) mice whereFcmr−/−(gray) serve as a negative control.b(Left) Dot plot illustrating peripheral blood CD11b + monocyte and neutrophil populations. (Right) Histogram overlay of Fcmr staining of peripheral blood innate immune cells inFcmr+/+(blue) mice whereFcmr−/−(gray) serve as a negative control.cDirect ELISA illustrating specific recognition of the extra-cellular domain of mouse Fcmr with in-house α-mouse-Fcmr antibody. Technical triplicates are represented with SE. Single-cell sequencing analysis Tumor mononuclear phagocytes (TMPs) were isolated via FACS and processed using standardized 10X Genomics Reagent Kit protocols. The raw sequenced reads were subjected to the CellRanger bioinformatics pipeline v2.0.1. The assembled UMI count matrix was processed using the Seurat R package v2.1.0 for quality filtering, normalization, clustering, and further downstream analyses. The final matrix contained counts for 16112 genes in 6352 Fcmr +/+ and 7999 Fcmr −/− cells. The expression-overlaid tSNE plots shown in Fig. 1 were produced using the FeaturePlots module of Seurat. The UMI histograms were produced using the raw UMI counts corresponding to the full set of cells before quality filtering. α-mouse Fcmr antibody Rat anti-mouse Fcmr sera were generated at an external vendor. In brief, four Lewis rats were immunized with purified recombinant mouse Fcmr-Fc protein [1] . After three subsequent immunizations of 0.1 mg each, serum was collected from each animal. To evaluate efficacy of rat immunization in producing specific and robust B cell responses to mouse-Fcmr, sera from these rats was used for ELISA and flow cytometry experiments. These data (Fig. 2 ) were subsequently used to inform on selection of two rats for splenic harvest and hybridoma generation. Although anti-Fcmr antibody titres were high in rat sera, this project ultimately failed to produce monoclonal antibodies of the desired affinity. Flow cytometry Peripheral blood was collected into heparinized capillary tubes via tail venipuncture and ejected into 5 ml polystyrene FACS tubes containing 100 μl PBS supplemented with 1% bovine serum albumin (BSA) plus 2 mM EDTA (referred to as FB buffer). Blood was collected from both Fcmr −/− mice and Fcmr +/+ , where Fcmr −/− served as the negative staining control. Peripheral blood in FB was pelleted at 300× g for 5 min at 4 °C, resuspended in 100 μl FB, and incubated for 10 min at 4 °C with 75 μl Fc Block (αCD16/32 2.4G2, Tonbo Bioscience; rat serum, StemCell) in FB containing DNase I (Roche). Rat polyclonal α-mouse-Fcmr was then added at a dilution factor of 1:100 and incubated for 30 min at 4 °C. Stained cells were washed via centrifugation in 2.5 ml FB at 300× g for 5 min at 4 °C, and resuspended in 100 μl Fc Block. 100 μl anti-rat secondary was then added to a final concentration of 1:200, and incubated for 30 min at 4 °C. Cells were again washed via centrifugation in 2.5 ml FB at 300× g for 5 min at 4 °C, resuspended in 100 μl FB, incubated for 10 min with 75 μl concentrated Fc Block. Following 10 min block, concentrated surface staining antibody cocktail (8x; 25 μl) [1] was added to a total volume of 200 μl and incubation continued for 30 min at 4 °C. Cells were again washed via centrifugation in 2.5 ml FB at 300× g for 5 min at 4 °C. Stained and washed whole blood was then subjected to fixation and red blood cell lysis. For this, pelleted whole blood from final wash was vortexed, resuspended in 1× Lyse/Fix Buffer (BD Biosciences, cat no. 558049), and incubated for 10 min. Cells were then pelleted (300× g for 10 min at 4 °C), supernatant discarded, and washed 2× via centrifugation at 300× g for 10 min at 4 °C with 2 ml FB. Cells were finally resuspended in 300 μl FB and analyzed by flow cytometry (Fortessa, BD Biosciences). ELISA Wells were coated with either mouse Fc (mFc), or mouse Fcmr-Fc (Toso-Fc) purified recombinant protein [1] , blocked, and washed. Rat polyclonal α-mouse-Fcmr was then added, incubated overnight at 4 °C. Plates were washed, incubated overnight at 4 °C with biotinylated α-rat secondary. Plates were again washed, and incubated with SA-HRP, washed, and bound antibody detected via TMB substrate. Plates were read at 450 nm.